A network approach for identifying and delimiting biogeographical regions Biogeographical regions (geographically distinct assemblages of species and communities) constitute a cornerstone for ecology, biogeography, evolution and conservation biology. Species turnover measures are often used to quantify spatial biodiversity patterns, but algorithms based on similarity can be sensitive to common sampling biases in species distribution data. Here we apply a community detection approach from network theory that incorporates complex, higher-order presence–absence patterns. We demonstrate the performance of the method by applying it to all amphibian species in the world (c. 6,100 species), all vascular plant species of the USA (c. 17,600) and a hypothetical data set containing a zone of biotic transition. In comparison with current methods, our approach tackles the challenges posed by transition zones and succeeds in retrieving a larger number of commonly recognized biogeographical regions. This method can be applied to generate objective, data-derived identification and delimitation of the world's biogeographical regions. Considerable attention has been devoted to develop methods that can confidently assign individuals to populations [1] , [2] , and then group those populations into phylogenetic entities that deserve the status of species or evolutionary units [3] . How species then co-exist and co-interact to form clusters at higher levels, of similar taxonomic and eco-physiological characteristics, is much less understood. This is surprising, considering that already by the 19th century prominent naturalists such as Humboldt and Bonpland [4] , de Candolle [5] , Prichard [6] , Sclater [7] and Wallace [8] had all realized that the world's biota is divided into a number of more or less distinct units. The recognition and use of biogeographical regions or bioregions, offers several advantages as compared with studying individual species or communities, and has therefore gained in popularity in recent years in both terrestrial and aquatic systems [9] , [10] , [11] , [12] . A bioregion-based approach in macroecology and evolution can be used to assess to what extent lineages are able to cross the major eco-physiological barriers over evolutionary time, that is, their degree of niche conservatism in a broad sense [13] , [14] . Evidence is growing that different bioregions will be affected differently by climate change [15] , [16] , so understanding their origins and evolution [17] , [18] may provide further indications of their expected resilience to future climate changes [19] . Bioregions may also be used as operational units in ancestral reconstruction analyses, aimed at inferring key biogeographical processes (dispersal, vicariance, speciation and extinction) for particular lineages [20] . Finally, a cross-taxonomic approach based on bioregions also offers important advantages in conservation biology as compared with focus on single taxa, not least in species rich areas such as seasonally dry tropical forests [21] , [22] . In such areas, conservational efforts may be better targeted towards protecting remaining patches of the threatened bioregions rather than focusing on particular species. In this sense, bioregions may be considered analogous to biodiversity hotspots, a concept based on species richness, endemicity and threat, which has received enormous attention in ecology, biogeography and conservation in the last decades [23] . Many studies take for granted the identity and delimitation of biogeographical regions around the world. Yet, there is little agreement on how to best classify and name such regions, with several conceptually related terms being used, often interchangeably [24] , [25] . These include biome, ecoregion, realm, province, zoo/phyto-geographic region, ecosystem, ecozone, chorotype, dominion, areas of endemism, concrete biota, chronofauna, nuclear area, horofauna, cenocron, phytocorion, generalized track, biogeographical/taxonomic/species assemblage and domain. Regionalization concepts vary among disciplines (for example, between zoology and botany) and regions, with for example, Africa having a generally accepted system for plants [26] , whereas South America lacks a unified, congruent floristic classification [22] , [27] . Moreover, different names may apply to the same unit; examples in South America include the Cerrado vs the Brazilian savanna, and the Páramo vs high altitude Andean grasslands (for an example see ref. 28 ). One common feature in most schemes of bioregionalization (the scientific discipline that deals with identifying, delimiting and naming biogeographical regions) is an internally implied hierarchy. This is for instance evident in the terrestrial classification system of Olson et al . [12] , which is the one adopted by the World Wide Fund for Nature (WWF) and recognizes eight realms, nesting 14 biomes which in turn contain 867 ecoregions. In that scheme, ecoregions are defined as ‘relatively large units of land containing a distinct assemblage of natural communities and species, with boundaries that approximate the original extent of natural communities prior to major land use change’ and reflecting ‘distributions of a broad range of fauna and flora across the entire planet’. This and other classification systems widely used in biogeography (for an example see ref. 8 ) include a key taxonomic component, thus contrasting with purely abiotic approaches such as the Köppen–Geiger Climate Classification [29] , which in its latest update [30] is based solely on ranges of temperature, precipitation and their distribution over the year. Perhaps more importantly than the lack of consensus in terminology and classification system used for biogeographical regions, which is to some extent more of a semantic issue rather than a true biological problem [25] , there remains controversy on how to best identify and delimit these regions—regardless of their hierarchical status. In the last decades, deductive approaches have started to be replaced by more analytical, transparent and reproducible methods [31] , [32] , [33] . However, bioregionalization based on species distribution data needs to deal with particular challenges such as biased taxonomic sampling. Even so, it has been shown to outperform even high-resolution remote sensing techniques that rely on structural differences in vegetation [22] and may therefore be more sensitive to human-mediated effects on the landscape, such as changes in land use and land cover (for example, clearing, plantations, irrigation, drainage and urbanization). The detection of bioregions is impacted by how we choose to quantify biogeographical structure, which up to now has been chiefly a variety of species turnover measures based theoretically on beta diversity [31] , [32] , [34] . Species turnover, as measured by set based similarity measures such as the Jaccard [35] , Sørenson [36] and β -similarity [34] , [37] , quantifies the relationship of one region to another, typically by dividing the number of shared species between two regions by some measure of the total species in both regions [38] . Despite their widespread use, species turnover measures can miss intricacies of distributional data that are relevant for bioregion detection. First, species turnover tends to increase with greater geographical distance from a source, bringing into question whether bioregions are determined by distance alone or real changes in taxonomic affinities [39] . Second, for small spatial scales the turnover can overestimate disparity due to competitive exclusion, spatial clustering and environmental gradients [40] . Although this problem can be reduced with large plot sizes, it is expected to persist even for large spatial scales. Furthermore, competitive exclusion can create geographical boundaries between species that cohabit the same bioregion. Third, some generally recognized bioregions span many degrees of latitude, such as the North American Rocky Mountains and the American Great Plains, and may contain climatic and environmental heterogeneities that can cause narrowly distributed taxa to occupy non-overlapping fractions of the same bioregion ( Fig. 1 ). Fourth, differences in taxonomic sampling are expected to inflate turnover. For example, taxonomic standards may differ within bioregions for rare species. For deep time studies, marine fossil assemblages may for instance not co-preserve aragonitic and calcitic shells. These processes collectively bias turnover measures, because the number of shared species cannot always be trusted as good gauge of bioregion identification. 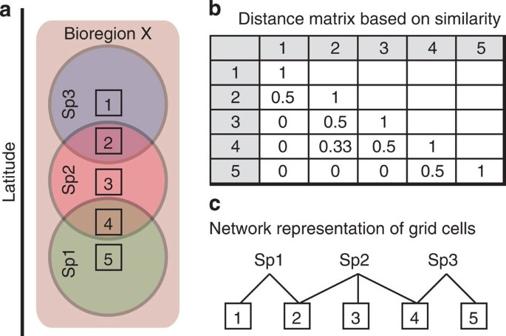Figure 1: Comparison between similarity based clustering and the network method. (a) Three species (Sp1, Sp2, Sp3) occur in the generally recognized Bioregion X, which spans a large latitudinal gradient. Species diversity is measured from five grid cells (numbered 1–5). Note that there is little geographical overlap between the species ranges, represented by circles. (b) Diversity similarity (set measures) between grid cells, which computes the similarity in number of shared species (the Jaccard index is shown here). Note that the distance between grid cell 1 and 5 is zero, since they do not share any species. (c) In the network method, connectivity between grid cells is established through the species they contain. In this case, grid cells 1 and 5 are ‘connected’ by a single step through one species (Sp2), which does not occur in either cell but occurs in other cells (2 and 4) occupied by species that also occur in cells 1 and 5 (Sp1 and Sp3, respectively). Figure 1: Comparison between similarity based clustering and the network method. ( a ) Three species (Sp1, Sp2, Sp3) occur in the generally recognized Bioregion X, which spans a large latitudinal gradient. Species diversity is measured from five grid cells (numbered 1–5). Note that there is little geographical overlap between the species ranges, represented by circles. ( b ) Diversity similarity (set measures) between grid cells, which computes the similarity in number of shared species (the Jaccard index is shown here). Note that the distance between grid cell 1 and 5 is zero, since they do not share any species. ( c ) In the network method, connectivity between grid cells is established through the species they contain. In this case, grid cells 1 and 5 are ‘connected’ by a single step through one species (Sp2), which does not occur in either cell but occurs in other cells (2 and 4) occupied by species that also occur in cells 1 and 5 (Sp1 and Sp3, respectively). Full size image Here we present a data-driven approach that uses associational networks to minimize the problems described above and to extract more community level information from species occurrence data. We show that this method can be used to successfully detect biogeographical regions in two well-validated empirical data sets: all amphibians of the world, and all vascular plants of the United States of America. The empirical data sets provide contrasting examples of how biodiversity data is currently available: they are aggregated at different scales (global and national), grain sizes (two degree grid cells versus US counties), and were constructed under different sampling methodologies. We then further validate our method on a hypothetical data set containing a zone of biotic transition. Our results are strikingly congruent with opinion based bioregions, indicating that the network method developed here holds the potential to greatly improve the identification and delimitation of the world's biogeographical regions. Amphibians of the world In an occurrence network ( Fig. 2a ), bioregions appear as groups of localities and taxa that are highly interconnected. 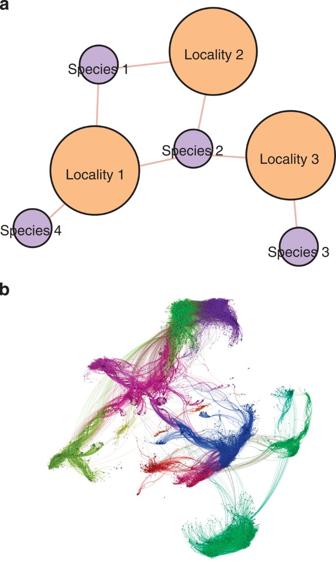Figure 2: Bipartite occurrence network. (a) Schematic representation showing the different classes of network connectivity that can be formed. Species 1 and 2 jointly occur in Locality 1 and 2, which creates a 4-path that loops, while Species 3 and 4 share a 4-path that does not loop, revealing that the species range of an intermediary species (Species 2) ‘connects’ the two. (b) A visualization of the global amphibian network analysed here (N=6,100 species). The geographical ranges of widespread species act as highways between biogeographical regions, creating links between clusters. Each cluster received a different, arbitrarily defined colour to increase contrast. Node positions were determined by the Force Atlas algorithm in the Gephi package66. Figure 2b shows a visualization of the network of all native amphibian species of the world. In this network, the broad spatial separations of clusters are closely equivalent to realms [8] , [33] , while the bioregions are coloured differently within each larger cluster. The links that cross between realms correspond to the relatively few widespread species that inhabit multiple bioregions on multiple realms and continents. Figure 2: Bipartite occurrence network. ( a ) Schematic representation showing the different classes of network connectivity that can be formed. Species 1 and 2 jointly occur in Locality 1 and 2, which creates a 4-path that loops, while Species 3 and 4 share a 4-path that does not loop, revealing that the species range of an intermediary species (Species 2) ‘connects’ the two. ( b ) A visualization of the global amphibian network analysed here ( N =6,100 species). The geographical ranges of widespread species act as highways between biogeographical regions, creating links between clusters. Each cluster received a different, arbitrarily defined colour to increase contrast. Node positions were determined by the Force Atlas algorithm in the Gephi package [66] . Full size image Our analysis identified 10 major bioregions (closely equivalent to zoogeographical realms) and 55 smaller biogeographical regions as the optimal representation of the full amphibian data set ( Fig. 3a ). This differs from the approach in Holt et al . [33] using a species turnover measure, which identified 19 bioregions as optimal. These results differ also qualitatively, showing some differences in the boundaries of the biogeographical regions detected. For instance, the network method is able to successfully detect Wallacea, a well known and thoroughly studied biogeographical region situated between Wallace's and Weber's line [41] , [42] (thick black lines in Fig. 3a ). Weber's line emerges as the major boundary between the Oceanian and Oriental faunas, corroborating the results by Holt et al . [33] which, however, did not recover Wallacea under the analysis of amphibian data. To illustrate how well range limits reflect bioregion structure, we coloured geographical ranges by the region they were assigned to ( Fig. 3b ). 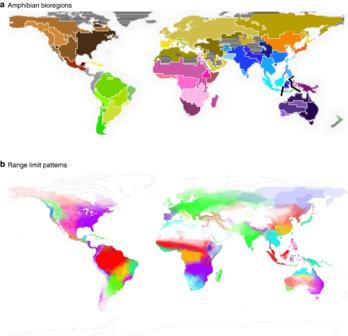Figure 3: Results from the network analyses for the world's amphibians. (a) Amphibian biogeographical regions of the world determined from geographical range data. Similar colours indicate membership to a higher level clustering, in this case equivalent to realms. The analysis used a resolution of two degree grid cells. (b) Species range limits coloured by region. Geographically close and neighbouring regions were given contrasting colours to highlight boundaries and boundary mixing. Each geographical range polygon was plotted with a low opacity (0.1), from largest to smallest on a global level, so that regions with more species appear brighter. (N=6,100 species). Figure 3: Results from the network analyses for the world's amphibians. ( a ) Amphibian biogeographical regions of the world determined from geographical range data. Similar colours indicate membership to a higher level clustering, in this case equivalent to realms. The analysis used a resolution of two degree grid cells. ( b ) Species range limits coloured by region. Geographically close and neighbouring regions were given contrasting colours to highlight boundaries and boundary mixing. Each geographical range polygon was plotted with a low opacity (0.1), from largest to smallest on a global level, so that regions with more species appear brighter. ( N =6,100 species). Full size image Vascular plants Comparing species turnover visually between different distance metrics is one way to build intuition about the differences between those metrics. Many network clustering methods do not use an explicit distance measure, but one can be derived to compare bipartite networks against the similarity approach. One such measure can be created as follows for the plant data: for a given focal county, extract its species occurrence list. Now, for each species in the occurrence list, give vote to each county that species i is distributed in, where n i is the number of counties that species i occupies. This builds a distance measure for the focal county against all other counties that share the focal county's species. 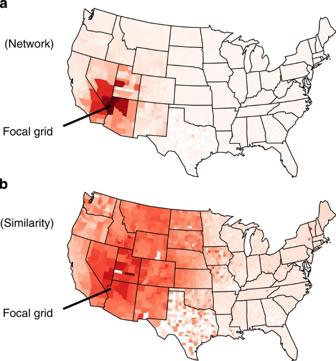Figure 4: Species turnover of vascular plants. Map of the USA showing how affinity decreases relative to an arbitrarily chosen county under (a) a network measure of distance and (b) a species similarity measure (hereβ-similarity). The colour gradient ranges from dark (high similarity) to light (low similarity). The network measure allows mid to narrow ranged species to contribute more strongly to the metric, revealing sharper boundaries of biogeographical regions. Figure 4 shows this approach applied to the plant data, revealing more localized distribution patterns than the similarity approach. We suggest this leads to a sharper delimitation of biogeographical regions ( Fig. 4a ) as compared with distributional data clustered by a similarity index, in which the taxonomic affinity of grids decreases gradually across space, diluting biogeographical signal ( Fig. 4b ). Figure 4: Species turnover of vascular plants. Map of the USA showing how affinity decreases relative to an arbitrarily chosen county under ( a ) a network measure of distance and ( b ) a species similarity measure (here β -similarity). The colour gradient ranges from dark (high similarity) to light (low similarity). The network measure allows mid to narrow ranged species to contribute more strongly to the metric, revealing sharper boundaries of biogeographical regions. Full size image Applying a commonly used similarity approach to our three United States Department of Agriculture (USDA) data sets of native plants, the number of clusters selected as optimal was 11 for all plants, 22 for trees and 14 for non-trees. The resulting optimal partition of counties for all data sets ( Fig. 5 , middle column) reveals little biogeographical structure. For all native plants, the boundary between the two largest clusters approximates the boundary between the American Great Plains and Eastern Temperate Forests, but it is dominated by rigid-state boundaries and fails to distinguish, for example, the Everglades in southern Florida, the Pacific Coast and the Rocky Mountains. The tree data set separates the Everglades from the rest of the United States, and the non-tree data set mimics the major boundaries in the data set with all plants but contains more clusters that are also US states. 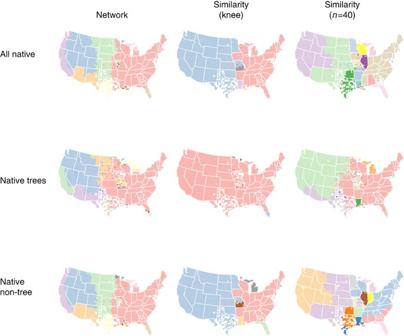Figure 5: Biogeographical regions of plants in the USA. The maps show demarcations for three subsets of the USDA plant database: all native plants, native trees, and native shrubs and herbs. The left column was determined by the map equation (under the optimal number of clusters in each analysis), while the middle and right columns were determined by a similarity approach (optimal number of clusters and an arbitrarily finer scale delineation, respectively). In each map, biogeographical regions were coloured differently to aid visualization (rather than reflect identify). Overall, the network approach captures with broad brushstrokes the patterns of the generally recognized biomes and biogeographical regions of the USA. Although state-level biases are apparent from both methodologies, they are strikingly more recurrent in the similarity approach. (N=17,600 species). Figure 5: Biogeographical regions of plants in the USA. The maps show demarcations for three subsets of the USDA plant database: all native plants, native trees, and native shrubs and herbs. The left column was determined by the map equation (under the optimal number of clusters in each analysis), while the middle and right columns were determined by a similarity approach (optimal number of clusters and an arbitrarily finer scale delineation, respectively). In each map, biogeographical regions were coloured differently to aid visualization (rather than reflect identify). Overall, the network approach captures with broad brushstrokes the patterns of the generally recognized biomes and biogeographical regions of the USA. Although state-level biases are apparent from both methodologies, they are strikingly more recurrent in the similarity approach. ( N =17,600 species). Full size image To explore whether the similarity approach could be arbitrarily forced to unveil deeper structure, we also chose to visualize the partitions with 40 clusters selected, although this delineation is not optimal ( Fig. 5 , right column). Some biogeographical structure becomes apparent at this level—the American Great Plains is cleanly separated from the American West, although this bioregion unrealistically extends into the American Southwest desert. The reconstruction based on these 40 clusters is also plagued by a number of boundaries coincident with the US state boundaries in the American midwest. In the tree level data, the Great Plains division becomes apparent, as well as a clean separation of the Southwest desert from the American West. In the non-tree data set, a latitudinal boundary is evident in the Eastern Temperate Forests bioregion, but also contains ample state-level biases. To test the application of our network method on vascular plants, we generated a network data set from the same USDA plant data, with county nodes connected to species nodes if the species was identified as natively present in that county. We clustered these data with the map equation—an algorithm that detects community patterns in networks [43] , [44] , [45] . A pilot analysis revealed little hierarchical structure in the data set, so we opted to use a two-level implementation of the map equation, which produces k clusters instead of hierarchically nested groups of clusters [43] . The apparent lack of hierarchy in the data set is likely an issue of large grain and low scale (counties within a single country). Higher-resolution data, such as a database produced from geographical coordinates, might produce greater subdivision. Applied to the three USDA data sets of native plants, the number of clusters selected as optimal by the map equation was 25 for all plants, 19 for trees and 16 for non-trees. Because the algorithm that seeks the best partition is stochastic, we ran it 1,000 times and selected the partition that minimized the scoring function in the map equation. Broad similarities are evident across the network clustering results for all native plants, trees and non-trees ( Fig. 5 , left column). There are, however, a number of differences. For instance, the Everglades are only evident from the tree only data set. The West Coast forms a separate bioregion under the analysis of all plants as well as all non-trees, but the Pacific Northwest is omitted from this bioregion when only trees are considered. In the American midwest, the American Great Plains appear much smaller when only trees are considered. These differences may reflect intrinsic biological differences among the data sets analysed (for example, differences in ecological niche conservatism, edaphic adaptations, dispersal ability), but sampling issues are also apparent. For instance, the southern deserts of Arizona and surrounding areas follow some rigid-state boundaries, suggesting that large county sizes in the area obscure finer demarcation. State-level biases are also evident in Lousiana for the native tree data, but not for the other two data sets. Hypothetical data set We compared the performance of the species turnover and the network approaches on a simulated data set. Using β -similarity and the unweighted pair group method with arithmetic mean on the hypothetical data set of Kreft and Jetz [46] , the transition zone is engulfed by the Northern realm for a choice of two clusters, and it is a distinct cluster if three clusters are chosen ( Fig. 6b ). The data are symmetric, so if the matrix rows are swapped the transition zone is engulfed by the Southern realm. 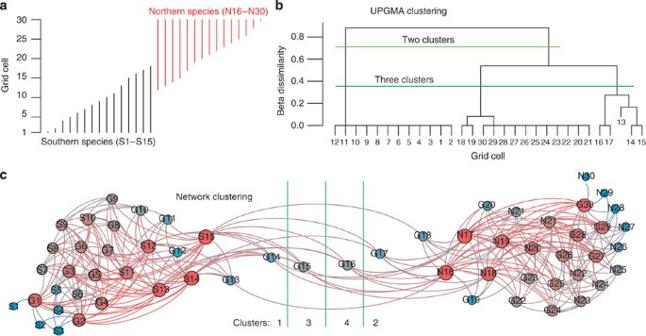Figure 6: Hypothetical transition zone. (a) Species range data across a line of grid cells. These data represent two biotic assemblages that blend together in a transition zone. (b) After clustering these data with the unweighted pair group method with arithmetic mean+β-similarity, the best representation of these data are as two or three clusters, but three clusters causes the transition zone to appear as a distinct biogeographical region. (c) In the network clustering, the best representation is as two or four clusters, with four being optimal (shown). In this optimal partition scheme, the transition zone is composed by two clusters, each containing a single species—correctly indicating that none of them can be confidently assigned to any of the major biotic assemblages. In the two cluster solution, the grid cells are divided evenly between the zones. Colours indicate the number of links that each node has: grid cells with higher richness and species with larger ranges are redder, while grid cells with less richness and species with smaller ranges are bluer. The sizes of the nodes are similarly proportional. ‘G’ denotes grid cell, ‘N’ denotes Northern species, and ‘S’ denotes Southern species. Node positions were determined with the Force Atlas algorithm in the Gephi software package66. (N=30 species). Figure 6: Hypothetical transition zone. ( a ) Species range data across a line of grid cells. These data represent two biotic assemblages that blend together in a transition zone. ( b ) After clustering these data with the unweighted pair group method with arithmetic mean+ β -similarity, the best representation of these data are as two or three clusters, but three clusters causes the transition zone to appear as a distinct biogeographical region. ( c ) In the network clustering, the best representation is as two or four clusters, with four being optimal (shown). In this optimal partition scheme, the transition zone is composed by two clusters, each containing a single species—correctly indicating that none of them can be confidently assigned to any of the major biotic assemblages. In the two cluster solution, the grid cells are divided evenly between the zones. Colours indicate the number of links that each node has: grid cells with higher richness and species with larger ranges are redder, while grid cells with less richness and species with smaller ranges are bluer. The sizes of the nodes are similarly proportional. ‘G’ denotes grid cell, ‘N’ denotes Northern species, and ‘S’ denotes Southern species. Node positions were determined with the Force Atlas algorithm in the Gephi software package [66] . ( N =30 species). Full size image Applying the network method to the same data results in an optimal partition of four clusters: one contains all of the Southern fauna and grid cells 1–14, one contains all of the Northern fauna and grid cells 17–30, while grid cells 15 and 16 each form their own cluster ( Fig. 6c ). This partition is slightly preferred over a two cluster solution, which cuts the data evenly into two biogeographical zones. This example reveals the benefit of clustering both species and grid cells together as under the network method, as opposed to clustering grid cells with distances proportional to the number of shared species; grid cells 15 and 16 can easily be identified as transition zones because no species are clustered with them ( Fig. 6c ). Our network analyses of empirical and hypothetical data sets reveal important differences as compared with approaches based on species similarity. These are not only quantitative in terms of resolution—that is, the total number of regions identified—but also qualitative, affecting both the areas and the boundaries of biogeographical regions. For the amphibian data set, the differences in number of zoogeographical realms and bioregions found by our network method as compared with the similarity analysis by Holt et al . [33] do not arise from a lower cutoff threshold for our approach, because we followed their procedure for merging regions with <10 grid cells into the closest regions. Rather, we interpret this difference as stemming from a fundamental difference in methodology—our approach clusters patterns of presence–absence relationships, while theirs identifies clusters of grid cells with low distributional and phylodistributional turnover. Our results suggest that, at least for amphibians, turnover measures based on species distribution data alone may be sufficient to identify realm boundaries. This conforms with the distribution only approach undertaken in Holt et al . [33] , which similarly identifies Weber's line as the realm boundary between the Oriental and Oceanian faunas, although it does not identify Wallace's line. This suggests that Weber's line may be more robust and independent of methodology than Wallace's line. At a finer scale, our analysis was able to recover many expert based biogeographical regions around the world. Taking South America as an example, our analysis not only identified the 2–3 major regions found by Holt et al . [33] , but also successfully recovered climatically and physiognomically distinct bioregions—roughly equivalent to biomes in WWF's classification [12] . These include the seasonally dry and fire prone Brazilian Cerrado, the evergreen Atlantic forest of eastern Brazil and the geologically old and nutrient poor Guianan highlands, among several other regions that were not recognized by our benchmark example using similarity [33] . We also note some important differences in the area and delimitation of these bioregions. The western limits of the Amazonian region inferred by Holt et al . [33] , for instance, cuts across the Andean mountains, despite the enormous altitudinal and physiological differences between these two regions. Our delimitations better conform to the commonly recognized boundaries between the Andes and Amazonia [47] , thus reflecting not only taxonomic differences but also current topography, climate and evolutionary history [48] . The inference of biogeographical regions for vascular plants of the United States of America led to similar methodological differences as compared with the analysis of amphibian data. In particular, the species clustering approach based on similarity exhibited both quantitative as well as qualitative shortcomings: it was unable to distinguish more than a few biogeographical regions under its optimal clustering, and it was heavily biased by political state boundaries ( Fig. 5 ). These shortcomings are perhaps unsurprising given a few challenges of the task, which we chose to illustrate the potential pitfalls encountered in empirical data sets of species distribution. First, we clustered raw occurrence data as presence or absence of a species in a county. This becomes evident in the output of the similarity analyses, as presence/absence data is often compiled at the state rather than the county level, producing apparently unique floras at the state level (mostly evident in Fig. 5 , right column). Second, county sizes differ substantially, creating an artifactual richness bias that is correlated with county size ( Supplementary Fig. 1 ). This pitfall might have been avoided by re-aggregating data by evenly sized grid cells and using an equal area coordinate system to remove latitudinal biases, but it should be already minimized by the Simpson's similarity index utilized. The compilation of spatial data under different aggregation schemes is well known to produce systematic biases in spatial analyses, a phenomenon termed the modifiable areal unit problem [49] , [50] . In cases where the taxa studied show clear geographical biases, such as American plants [51] , species distribution models (SDMs) could have been used as an alternative to range maps. This would have reduced the bias of identifying political state boundaries as bioregion limits in our empirical example using the similarity approach ( Fig. 5 ). However, we identify two inherent pitfalls. First, SDMs are still largely sensitive to the data and methodology used [52] , carrying their own sets of problems and assumptions—such as reliance on interpolated climatic data, general unavailability of non climatic niche variables and exclusion of potentially crucial lineage-specific traits such as dispersal ability, biotic interactions, population dynamics and evolutionary history [53] . Second, using SDMs for bioregion inference could become conceptually circular. If we are to understand how species cluster into distinct bioregions, and how the boundaries of these bioregions relate to environmental gradients, this comparison needs to be post hoc . We cannot use SDMs to delineate the same bioregions that are then used to compare their correspondence with the environmental variables, because these variables are already the major component of SDMs. Considering these pitfalls, we argue that new methods for biogeographical delineation must be designed around the current challenges offered by real occurrence data—which are geographically and taxonomically biased, but nevertheless constitute the most reliable evidence on where species occur. Here we have provided evidence that the network approach presented here outperforms the current methods based on similarity. In conclusion, the tendency of species to remain in their optimal environment over evolutionary time has been suggested as a crucial feature shaping the uneven distribution of the world's biota [13] , [18] , [54] , including the establishment and maintenance of the tropical gradient in species richness. The origin and evolution of bioregions is also gaining focus in macroecological meta-analyses using phylogenetic, palaeontological and distribution data [14] , [33] , [48] . Phylogenetic turnover measures have been used as alternative to [55] , as well as in combination with [13] , species distribution data. However, they rely on robust and well-sampled species-level phylogenies (which are currently lacking for many organismal groups) and may introduce circularity when using the identified bioregions for measuring the degree of phylogenetic niche conservatism as shifts in bioregions are commonly associated with speciation events. Phylogenies, especially when time calibrated, can be subsequently used to shed light on the temporal origin, evolution and phylogenetic relatedness of bioregions. Important challenges, however, remain in order to further advance bioregionalizations: 1 Quantity and quality of species occurrence data. Mapping the distribution of the world s estimated 8.7 million species [56] constitutes a major challenge in biological research [57] and is paramount for bioregion delineation. The ever increasing digitization of natural history collections worldwide now offers access to over 500 million records at the Global Biodiversity Information Facility ( www.gbif.org ), but this figure is still far from the estimated total of one billion specimens. It is clear that the occurrence data currently available contain substantial spatial, taxonomic and temporal biases [58] , besides a certain proportion of errors (for example, misidentified specimens and poorly or wrongly annotated locality information). Substantial efforts are required to revise such raw occurrence data and combine them with field observations and expert knowledge, for producing GIS based polygons of species distribution ranges (for example, IUCN and Map of Life, http://mol.org ). 2 Methodological development and integration. Bioregionalization will greatly profit from bringing together different techniques, data and disciplines. These could include remote sensing, climatic mapping and bioregion modelling based on key species [22] . New methodologies for bioregion delineation need to be reproducible and transparent about their assumptions. They should offer measures of reliability regarding the number and boundaries of species clusters identified, for example through bootstrapping techniques. In some cases, the delimitation of the same bioregion may be more or less robust along different edges. Finally, they should be regularly validated through ground truthing. 3 Theory versus reality. Are biogeographical regions real and natural entities, how were they formed, how are they maintained through time and space? We still lack an elementary ecological theory for addressing these questions, despite the fact that few people contest their existence. We also need to understand how extrinsic (for example, climate, geological history and soils) and intrinsic (for example, functional traits, biotic interactions and physiology) variables interplay to produce the differences we observe in the number and delimitation of bioregions based on data from plants, birds, amphibians and mammals (ref. 33 and this study) and expand our inferences to many other understudied groups. More than a century after the first biogeographical regions were proposed [8] , we may now have enough data to delimit the world's biogeographical regions in greater detail than Wallace could ever envision. Our study, however, illustrates that new methodologies play a crucial role in this process and that network methods offer a new set of exciting tools to classify, delimit and better understand biodiversity. Delimiting bioregions with networks To classify bioregions based on species distribution data we hierarchically classify groups of species and grid cells into biogeographical regions. To achieve this goal we borrow from the techniques developed in network science to create a network that will be meaningful for biogeographical analyses, and then use network clustering algorithms to hierarchically partition the groups of nodes into clusters. In this paper we adapt the methodology presented by Vilhena et al . [59] and Sidor et al . [45] for modelling species distributions as a network. We first build the network to be clustered, and then we choose the best clustering algorithm to infer bioregions. A bipartite network ( Fig. 2 ) has two disjoint sets of nodes with no links between nodes of the same set. Many biological systems have been abstracted as bipartite networks, such as plant-pollinator interactions inferred by visitation [60] , sexual contact between heterosexual partners [61] and interactions between prey and bait proteins generated by yeast two-hybrid screening, an experimental method to test whether pairs of proteins interact [62] . Geographical relationships between species and localities can also be abstracted as a bipartite association network, where links are the occurrences of species within geographical locations. Interpretations derived from analyses of presence–absence networks are comparable with plant-pollinator networks, because relationships between entities of the same set are associational, such as co-visitation and co-occurrence. Second-order relationships in presence–absence networks are paths of length two or 2-paths. The number of 2-paths between species is the number of times those species co-occur, while the number of 2-paths between a pair of localities, regions or grid cells is the number of species shared by both the grid cells. Although second-order range overlaps between two species may not be directly intuitive biologically, in practice it should allow the delimitation of bioregions comprised of only partially overlapping species. Partial occupancy of a species' potential range ( Fig. 1a ) may be due to intrinsic traits (for example, dispersal ability, tolerance to specific climatic and environmental variables, ecological interactions) as well as the region's physical features (for example, soil and climatic heterogeneity, geological history, presence of dispersal barriers). A more complicated pattern is the number of joint occurrences, where two species occupy the same two localities. This can be measured as the number of four paths that complete a loop ( Fig. 2a ). These relationships can be combined to reveal properties of geographical ranges. For example, the number of 3-paths between a species A and locality B divided by the number of 2-paths exiting from species A is the fraction of co-occurrences of species A that also occupy locality B. By setting up the machinery to capture ‘higher-order’ patterns, we can detect complex patterns of presence-absence. The adjacency matrix A of this network formally expresses species occurrences, and is written For the rows and columns of this matrix, we order first by species (1... n ) and second by grid cells ( n + 1... n + m ), producing a square matrix with n + m rows and n + m columns. This is expressed where B is the binary presence–absence matrix, in which rows are taxa and columns are localities. The upper left block and lower right block in this matrix are zeroes, because species cannot occur in species and localities cannot occur in localities. The square of the adjacency matrix A gives the co-occurrence matrix C between taxa as the upper left square, or number of co-occurrences between pairs of species, and the matrix of shared species S as the bottom right square or number of shared species between the pairs of grid cells where elements in the upper right and lower left squares of the matrix are zeroes because 2-paths are exclusively between two species or between two localities. Total paths of length i between nodes can be expressed by raising the matrix to the i th power. By formulating the data in this way, new measures can be derived and tools from network theory can be readily applied. In the next section we apply a common clustering algorithm to this bipartite network. Clustering the bipartite species network Among candidate clustering algorithms, the map equation is the most suitable approach to be extended to bipartite networks [43] , [44] , [45] . The map equation is a general approach that, for our purposes, corresponds to an intuitive process. First, the algorithm chooses a random grid cell. It then randomly chooses a species found in that grid cell, examines the geographical range of that species, and selects a grid cell at random within its geographical range. It repeats this process iteratively and exhaustively. In biota with substantial biogeographical structure, the algorithm would spend long time intervals within bioregions, crossing only when it selected a cross-bioregion species. If the algorithm would be requested to report a list of the grid cells and species chosen, it would save time to simply list the bioregions visited. The map equation quantifies the tradeoff between losing detail from all visits and saving time by communicating a shorter list; in biota with strong biogeographical structure, it will be better on average to communicate a shorter list of visits. The map equation has been extended to deal with hierarchical partitions, which we use to reveal biogeographical regions [43] , [44] . The software packages for the two level and hierarchical approaches are available online ( http://www.mapequation.org ). Method validation and performance As a first empirical test case, we apply the network clustering method to the International Union for Conservation of Nature (IUCN) amphibian database, which contains range shape files for each of the world's c. 6,100 included species. We use only native ranges for the analysis. We choose to analyse distributional data for amphibians [63] because (i) we consider this database to be thoroughly verified by the scientific community; (ii) we expect that the eco-physiological tolerance of amphibians should be narrower than for example that for mammmals or birds, and therefore more closely represent generally recognized biogeographical regions; and (iii) this would allow a direct comparison with a recent study by Holt et al . [33] , where both the species distribution data alone and combined with phylogenetic information was used to infer zoogeographical regions and realms at a global scale. Our second empirical test is performed using the USDA plant database, which contains the presence or absence of 22,918 native vascular plant taxa (corresponding to 17,600 species) spread through 50 states and 3,143 counties of the USA. We use only the range of native plants, delineating bioregion structure for all plants, only trees and all plants except trees (that is, herbs, lianas, shrubs, subshrubs and vines). These data are ideal as a benchmark because they contain several challenges for computational methods. First, the United States county areas are longitudinally biased, with larger counties in the west and smaller counties in the east ( Supplementary Fig. 1 ). Second, plant distributions are aggregated differently across the states, causing systematic compositional biases across state borders. Third, counties are unevenly sampled. To our knowledge, no quantitative bioregion delineation of these data are available for direct comparison. Finally, we use a recent hypothetical data set to illustrate key differences between our network method and species similarity approaches. In a recent commentary by Kreft and Jetz [46] , this data set was created to showcase potential pitfalls for selecting the wrong number of clusters. The hypothetical data contains a transition zone, where the most widespread species in a Northern and Southern biota co-occur ( Fig. 6a ). In their analysis [46] , the number of clusters selected as optimal was shown to fully determine whether or not the transition zone appeared as distinct biogeographical regions. This result was used to illustrate the danger of classifying transition zones as distinct biogeographical regions, but also highlights the sensitivity of inferring biogeographical regions based on species similarity measures. To assess the performance of our network-based clustering with a conventional species similarity approach, we opted for the methodology selected as best in a recent methods review by Kreft and Jetz [32] . To apply that approach to our plant data, we created a matrix of counties and computed the species similarity between each pair of the US counties with species data. We applied the β sim index to the different data sets, written . Here a is the number of shared species between two species assemblages and b and c are the total unique species to either assemblage (quadrat, locality, grid cell and so on). Note that β sim is 0 when the species assemblages are either identical or the smaller assemblage is a subset of the larger assemblage, and β sim is 1 when the assemblages contain no shared species. This measure is considered ideal over more conventional measures (such as the Jaccard) because it is less sensitive to differences in species richness [32] . To further illustrate how the network measure compares with β -similarity, we calculated taxonomic plant similarity between each US county and an arbitrarily selected focal grid (the Mohave County in Arizona), following a similar methodology as described in previous studies [10] , [32] , [64] . We then performed the same calculation using the network measure and projected the results on a map. Finally, we clustered the full species similarity matrix with the unweighted pair group method with arithmetic mean approach to generate a hierarchical dendrogram that summarizes the distances between counties. From this dendrogram, we selected an optimum number of clusters by finding the ‘knee’ in the evaluation curve [65] , with the average percentage of county level endemics as our evaluation measure [32] . How to cite this article: Vilhena, D. A. and Antonelli A. A network approach for identifying and delimiting biogeographical regions. Nat. Commun. 6:6848 doi: 10.1038/ncomms7848 (2015).